Carbon prospecting in tropical forests for climate change mitigation Carbon finance projects that protect tropical forests could support both nature conservation and climate change mitigation goals. Global demand for nature-based carbon credits is outpacing their supply, due partly to gaps in knowledge needed to inform and prioritize investment decisions. Here, we show that at current carbon market prices the protection of tropical forests can generate investible carbon amounting to 1.8 (±1.1) GtCO 2 e yr −1 globally. We further show that financially viable carbon projects could generate return-on-investment amounting to $46.0b y −1 in net present value (Asia-Pacific: $24.6b y −1 ; Americas: $19.1b y −1 ; Africa: $2.4b y −1 ). However, we also find that ~80% (1.24 billion ha) of forest carbon sites would be financially unviable for failing to break even over the project lifetime. From a conservation perspective, unless carbon prices increase in the future, it is imperative to implement other conservation interventions, in addition to carbon finance, to safeguard carbon stocks and biodiversity in vulnerable forests. Nature-based solutions could contribute substantially to climate change mitigation [1] , [2] . These solutions include the protection, restoration, and improved management of forests, wetlands, grasslands, and agricultural lands to increase carbon dioxide sequestration, reduce emissions and enhance climate resilience [1] , [3] . Protecting and ensuring the health of natural ecosystems are also important for conserving biodiversity, providing clean air and water, safeguarding food security, and sustaining livelihoods [1] , [4] . The climate mitigation potential and co-benefits of nature-based climate solutions, in turn, present exciting opportunities for the public and private sectors to meet their climate goals, invest in carbon finance, and contribute to addressing the impacts of climate change [5] , [6] . Indeed, with increasing support and interest from institutions such as the World Bank, the transacted volume of nature-based carbon credits in the voluntary carbon market grew by over 250% between 2016 and 2018, from 14 MtCO 2 e to 51 MtCO 2 e [6] . The growing demand for high quality, nature-based carbon credits may be outpacing their supply [6] , [7] , as indicated by a 30% (or $1.1 t −1 CO 2 e) increase in the average price of carbon offsets associated with nature-based solutions in 2019 compared to the previous year [7] . The bottleneck in shovel-ready carbon projects may be due in part to gaps in knowledge critical for supporting and informing investment decisions on both protecting existing carbon stocks (e.g., avoided deforestation) and enhancing new carbon stocks (e.g., reforestation). For example, while the protection of tropical forests could in principle contribute substantially to climate mitigation by safeguarding their forest carbon [8] , these carbon stocks may not all be fundable through carbon finance, and hence not all be investible. In fact, only the subset of forest carbon stocks that are under imminent threat of decline or loss if left unprotected by a conservation intervention may be certifiable [9] , [10] . This criterion of ‘additionality’ is a pre-condition for certifying all carbon credits, including nature-based credits traded in the voluntary carbon market, under the rules of the United Nations Framework Convention on Climate Change and reducing emissions from deforestation and forest degradation (REDD) and REDD + programmes [9] , [11] . We modeled the magnitude of certifiable carbon from forest protection projects (hereafter referred to as ‘investible forest carbon’), and its climate mitigation potential to produce a global investible forest carbon map at 1-km resolution (Fig. 1 ). We achieved this by analyzing the spatial distribution of existing forest carbon stocks [12] , with respect to their projected future risk of deforestation to account for additionality [13] , while also incorporating other key criteria of the Voluntary Carbon Standard (VCS) [9] (see Methods for details). Fig. 1: Global investible forest carbon across the tropics. The estimated volume of investible carbon from the five countries with the highest potential in each of the tropical regions of the Americas, Africa, and Asia-Pacific are highlighted. Full size image Investible forest carbon Our analysis shows that the protection of tropical forests worldwide could generate investible carbon amounting to 1.8 (±1.1) GtCO2e yr −1 (Fig. 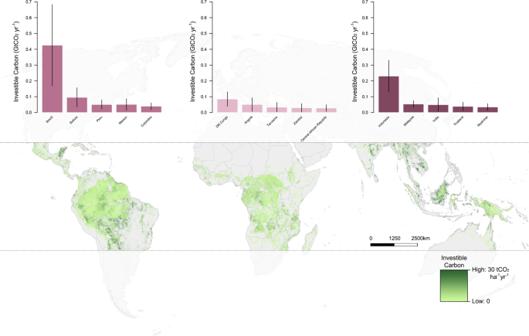Fig. 1: Global investible forest carbon across the tropics. The estimated volume of investible carbon from the five countries with the highest potential in each of the tropical regions of the Americas, Africa, and Asia-Pacific are highlighted. 1 ; Table 1 ). Much of this carbon would originate from the Americas (809.1 ± 487.7 MtCO 2 yr −1 ) and the Asia-Pacific region (581.8 ± 311.8 MtCO 2 yr −1 ). The African continent has substantially lower potential for generating investible carbon from tropical forest projects (392.7 ± 286.5 MtCO 2 yr −1 ). These findings are important to both potential investors of new forest protection carbon projects and local forest stakeholders for highlighting opportunities to generate revenue from carbon projects as an alternative to the business-as-usual scenario of destroying these forests. Table 1 Global, regional, and country-level estimates of investible carbon and return-on-investment (based on net present value). Full size table Our estimates of investible forest carbon are ~31% lower than those reported in previous studies [1] , [3] , which were largely based on aggregated country level data on carbon stocks and deforestation rates. Furthermore, our analysis also incorporates VCS criteria, such as the requirement to set aside buffer credits [9] , not considered in other studies [1] , [3] . As such, we are able to compare our estimates of investible forest carbon with actual volumes of verified carbon units (VCUs) reported by 25 real-world VCS projects on forest protection across the tropics. We achieved that based on empirical VCS data, including 111 ground-based and verified carbon stock measurements from projects across 16 countries. We find a relatively strong correlation ( R = 0.49, p < 0.05) and no significant difference ( t = 0.92, p = 0.36) between our estimates and the ground-based measurements of verified carbon units (Fig. S1 ). Globally, the top five countries in terms of investible carbon are Brazil (426.2 ± 257.0 MtCO 2 yr −1 ), Indonesia (230.5 ± 99.7 MtCO 2 yr −1 ), Bolivia (96.0 ± 60.8 MtCO 2 yr −1 ), Democratic Republic of Congo (85.3 ± 45.3 MtCO 2 yr −1 ) and Malaysia (53.6 ± 21.4 MtCO 2 yr −1 ) (Fig. 1 ; Table 1 ). Barriers to the establishment of forest carbon projects may include competing interests and priorities from other economic sectors (e.g., agriculture), lack of enabling conditions and policies, governance and institutional constraints, and prohibitively high technical entry bar [14] , [15] , [16] . Such barriers can further limit the potential of forest protection as a nature-based climate solution when compared to other forestry and forest restoration based techniques [17] , [18] . Many of these barriers may be overcome if actionable information regarding both the financial risks and return-on-investment of projects is available to incentivize solutions. Financially viable forest carbon Indeed, investible carbon projects may not all be profitable. The financial viability of a project depends on a range of factors, including operational costs and carbon pricing, as well as political risk, which may vary with location and over time [19] . We modeled the relative profitability of these projects to produce a global forest carbon return-on-investment map (Fig. 2 ). Fig. 2: Global forest carbon return-on-investment from financially viable sites. Estimates are presented as net present values over a 30-year timeframe, highlighting the corresponding estimates across each region and five countries with the highest potential. We also present the accumulation of profits overtime at the global and regional levels, with shadings around the lines representing standard deviation (inset). Full size image We based our analysis on several simplifying assumptions (see Methods for details). Briefly, we applied a cost estimate of $25 ha −1 for project establishment, and $10 ha −1 y −1 for subsequent years for project maintenance. We also assumed a constant carbon price of $5.8 t −1 CO 2 for the first five years, followed by a 5% price appreciation for the subsequent years over a project timeframe of 30 years [19] . Finally, we applied a risk-adjusted discount rate of 10% in our calculation of net present values (NPV) for the return-on-investment of tropical forest carbon projects [20] , [21] . We find that the vast majority of financially viable (i.e., yielding positive NPV) and most profitable forest carbon sites (>$308 ha −1 y −1 ; 90th percentile) are located in the Asia-Pacific region with NPV amounting to $24.6b y −1 , compared to the Americas ($19.1b y −1 ) and Africa ($2.4b y −1 ) (Fig. 2 & S2 ; Table 1 ). This largely reflects the fact that tropical forests in the Asia-Pacific region both contain high carbon density and are facing high deforestation risks, thereby creating immense opportunities for avoiding carbon emissions through forest protection [22] . Of course, the high risk of deforestation may also pose a challenge to the long-term environmental integrity of these projects, which also needs to be considered and mitigated through other national or region-specific policy measures. The top five countries with highest return-on-investment are Brazil ($11.2b y −1 ), Indonesia ($10.1b y −1 ), Malaysia ($2.6b y −1 ), Bolivia ($2.5b y −1 ) and India ($1.7b y −1 ) (Fig. 2 & S2 ; Table 1 ). This represents a substantial amount of potential returns from the trading of carbon credits in markets that could support the protection of forests, thereby benefiting forest stakeholders. Globally, ~80% (1.24 billion ha) of the investible forest carbon sites would be financially unviable for carbon finance for failing to break even over the project lifetime (i.e., yielding negative NPV; Fig. 2 ). Importantly, these forests represent forgone climate mitigation at a rate of 0.7 GtCO 2 yr −1 , assuming no other conservation measures are taken. From a forest conservation perspective, these findings suggest that carbon finance will fail to protect the vast majority of investible carbon sites, which are also, by definition, vulnerable to deforestation (Fig. 2 & S2 ; Table 1 ). However, if global demands for nature-based carbon credits continue to grow [6] , future carbon prices may also increase. We modeled the effects of carbon pricing on the financial viability of forest carbon sites globally. We find that at a global level, carbon pricing at $16 t −1 CO 2 and $44 t −1 CO 2 are needed to protect 50 and 80% of investible carbon sites, respectively (Fig. 3 ). Further carbon price increases above $50 t −1 CO 2 would only bring marginal forest conservation and climate mitigation benefits (Fig. 3 ). We also find that this sensitivity to carbon pricing varies geographically. For example, carbon prices of $7.1 t −1 CO 2 for Asia-Pacific, $17.2 t −1 CO 2 for the Americas, and $17.7 t −1 CO 2 for Africa, are needed to protect 50% of the investible forest carbon sites in these respective regions (Fig. 3 ). These carbon prices may be potentially achievable in the near future, given the growing global interest in nature-based carbon credits, and suggests that carbon pricing may be an important lever to drive investments for nature-based climate solutions through carbon finance [6] , [7] . Fig. 3: Effect of carbon pricing on the financial viability of forest carbon sites. Graph indicates the proportion of investible forest carbon that are financially viable for carbon finance. Shadings around the lines represent confidence bands based on standard deviation. Full size image However, in the same way that carbon pricing can affect the financial viability of forest carbon projects, so too can changes in the operating expenses of these projects. In a separate analysis, we find that increases in the establishment and annual maintenance costs by 50% and 100% would result in decreases in the global volumes of profitable forest carbon by 19.6% to 892.1 ± 559.2 MtCO 2 yr −1 and 34.3% to 728.8 ± 462.2 MtCO 2 yr −1 , respectively (see Methods; Table S1 ). Furthermore, it is also important to note that some financially viable but less profitable forest carbon sites will struggle to compete with lucrative land uses, particularly in countries such as Brazil and Indonesia, which are the world’s major producers of soy, beef, and palm oil [19] . In other countries, such as the Democratic Republic of the Congo, hydrocarbon exploration and logging developments with multiple vested interests may pose additional barriers to carbon projects [23] . To understand the potential impacts of these opportunity costs, we performed another separate analysis that takes into account the land rent from potential agricultural and forestry developments that may compete with forest carbon projects (see Methods). We find when all forests are excluded where opportunity costs are higher than returns from carbon finance, the global climate mitigation potential of forest protection would decrease by 47.7% to 580.6 ± 368.6 MtCO 2 yr −1 (Table S1 ). Therefore, it is imperative to implement other conservation strategies and interventions to safeguard the carbon stocks and biodiversity in these vulnerable forests. Critically, carbon finance must be placed in the broader context of other incentives and policies targeting both the corporate and government sectors to protect forests and avoid emissions. An example is Costa Rica’s model of using part of their carbon tax revenue to support the protection and restoration of natural ecosystems across the country, with direct payments made to farmers and landowners for their compliance [24] . Obviously, there is a wide range of environmental, socioeconomic, governance, and geopolitical factors that can influence climate strategies, conservation actions, and investment decisions [25] . For example, some carbon projects may include financially unviable sites that are important for conserving biodiversity, safeguarding rural livelihoods, or providing other co-benefits that may be highly valued by society but not internalized in our analysis [4] . Such financially unviable sites could potentially become viable by leveraging on payment schemes for other ecosystem services beyond carbon storage. Furthermore, the political ecology landscape of existing and new carbon investments within a host country may also influence and alter the risk of deforestation, which affects additionality, the long-term success of forest carbon projects, and ultimately the permanence of carbon credits or the diversion of development and deforestation to other locations (i.e., leakage effects) [10] , [11] . For example, the political risk for certified carbon credits has recently increased significantly in Brazil. In exchange for political support, the Brazilian government laid the foundation for landowners to accelerate deforestation [26] . This political bargaining may have seriously compromised Brazil’s ability to meet the Paris target. These political risk considerations are crucial to ensure the long-term viability of carbon investments. One approach to mitigate the risks of non-permanence and leakage effects of forest carbon projects is to require project developers to set aside buffer credits, which is in fact already a requirement under the VCS (i.e., requiring 20% of total credits to be set aside as buffer). We find that if this requirement is increased by an additional 10%, 20%, or 30% will decrease the global volume of profitable forest carbon by 18.1% to 909.1 ± 567.4 MtCO 2 yr −1 , 35.4% to 716.7 ± 448.4 MtCO 2 yr −1 or 51.7% to 535.8 ± 336.3 MtCO 2 yr −1 , respectively (see Methods; Table S1 ). Our analyses draw from a sliver of the best available data to provide a snapshot of the relative investible carbon and return-on-investment for the protection of tropical forests as a nature-based climate solution. While we find that carbon finance may fail to protect a large proportion of tropical forests at current carbon prices, nature-based climate solutions remain hugely important for the many other co-benefits they provide for society. By clarifying some of these opportunities and constraints, we help to calibrate expectations and incentivize public and private sector investments in nature-based climate solutions to benefit the environment, climate, and society. Overview of methods First, we modeled and mapped investible forest carbon, and its climate mitigation potential across the tropics at 1-km resolution. Second, we compared our estimates of investible forest carbon with actual volumes of VCUs reported by 25 real-world VCS forest protection projects. Third, we modeled the relative profitability of investible forest carbon sites to produce a global forest carbon return-on-investment map based on their NPV. All calculations were based on data dated between 2012 and 2017 and at a resolution of 0.00833 degrees (~1 km). To ensure data standardization, we resampled (bilinear) finer-scaled data where necessary, for example, for data sourced from the European Space Agency - Climate Change Initiative -Land Cover [27] . We only considered tropical forests between ~23.44°N and 23.44°S, and excluded all land cover types that would preclude forests, for example, savannas, bare ground, water, agriculture and urban areas [27] . Investible forest carbon We first estimated the total volume of CO 2 associated with three carbon pools in tropical forests: aboveground carbon, belowground carbon, and soil organic carbon. Next, we applied key VCS criteria, including additionality, to model and map investible forest carbon across the tropics. Mapping total volume of CO 2 associated with tropical forests Aboveground carbon We applied a stoichiometric factor of 0.475 to recent spatial data on aboveground carbon biomass [12] (i.e., for period 2012–2016), to convert it from biomass to carbon stock values, based on established carbon accounting methodology [3] , [28] , [29] . We performed an uncertainty analysis to account for potential variability in this stoichiometric factor (see ‘Uncertainty analysis’ section below). We applied a conversion factor of 3.67 to derive the volume of CO 2 associated with this carbon pool [3] . Belowground carbon We derived belowground carbon biomass by applying two different allometric equations relating root to shoot biomass [30] to the most recent spatial dataset on aboveground carbon biomass [12] , following established carbon accounting methodology [3] , [28] , [29] . The two equations are: belowground biomass = 0.489 × aboveground biomass^0.89; and belowground biomass = 0.26 × aboveground biomass. We then applied a stoichiometric factor of 0.475 to the estimated belowground carbon biomass to convert it from biomass to carbon stock values. Next, we calculated the mean, minimum and maximum values for belowground carbon based on an uncertainty analysis (see ‘Uncertainty analysis’ section below). We applied a conversion factor of 3.67 to derive the volume of CO 2 associated with this carbon pool [3] . Soil organic carbon We also considered soil carbon due to its potentially significant contributions to carbon storage [31] and despite potential uncertainties and variability surrounding its measurements [32] . Specifically, we utilized the organic carbon density of the topsoil layer (0–30 cm) obtained from the European Soil Data Centre [33] as it represented the best data available of soil organic carbon. We applied a conversion factor of 3.67 to derive the volume of CO 2 associated with this carbon pool [3] . Applying VCS criteria to map investible forest carbon The criterion of additionality is a pre-condition for certifying all carbon credits under the VCS. This implies that only the volume of forest carbon that are under imminent threat of decline or loss if left unprotected by a conservation intervention can be certified under the VCS. We derived the volume of forest carbon under threat of loss based on best available proxy data on projected future deforestation rates across the tropics [13] (through to the year 2029), and annualized over the prediction period (15 years). We applied this estimated annual deforestation rate to the total volume of CO 2 associated with tropical forests as estimated above, to derive the volume of CO 2 that would be certifiable and therefore investible under the VCS. 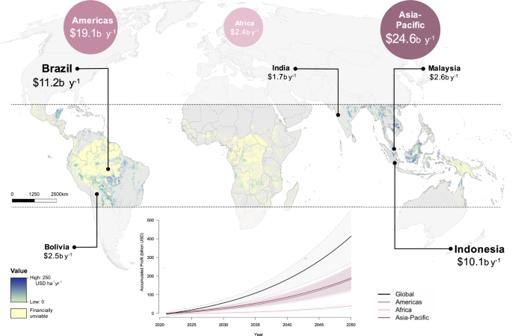Fig. 2: Global forest carbon return-on-investment from financially viable sites. Estimates are presented as net present values over a 30-year timeframe, highlighting the corresponding estimates across each region and five countries with the highest potential. We also present the accumulation of profits overtime at the global and regional levels, with shadings around the lines representing standard deviation (inset). 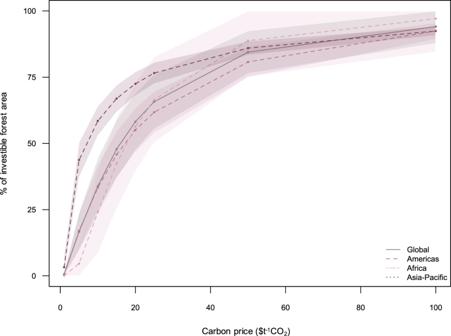Fig. 3: Effect of carbon pricing on the financial viability of forest carbon sites. Graph indicates the proportion of investible forest carbon that are financially viable for carbon finance. Shadings around the lines represent confidence bands based on standard deviation. We also assumed a conservative 10-year decay estimate for the belowground carbon pool [9] . Additionally, we excluded lands that will likely not be certifiable for other reasons [9] , including recently deforested areas [34] (i.e., for the period 2010–2017), as well as human settlements located within these forests [35] . Lastly, we accounted for the VCS requirement to set aside buffer credits of 20% to account for the risk of non-permanence associated with Agriculture, Forestry and Other Land Use projects (AFOLU) [9] . Comparing estimates of investible forest carbon to verified carbon units We compared our estimates of investible forest carbon with actual volumes of VCUs reported by real-world VCS forest protection projects ( https://verra.org/ ). We identified a set of 25 VCS forest protection projects from across 16 countries that met the following criteria: ii) includes spatial data on project boundary in their project documentation; ii) the project extent is located entirely within the tropics; and 3) has been verified (i.e., either “verified, under verification” or “verification approve”) (Table S2 ). We extracted the shapefiles (i.e., geometric polygons) of these VCS projects, and overlay them on our map of investible forest carbon to extract the volume of investible forest carbon (CO 2 ) from our analysis that corresponds to each of the 25 VCS forest project. We then compared our estimates of investible forest carbon to the volume of VCUs issued between 2005 and 2018 for each VCS project. The number of data points reported per year for each project ranged from 1–10, and generated a total of 111 data points for comparison. We then assessed the degree of correlation (i.e., Pearson’s correlation), relative accuracy (i.e., Root Mean Square Error; RMSE), and statistical difference (i.e., paired t-test) between the two datasets. Estimating return-on-investment Based on our map of investible forest carbon, we modeled the relative profitability of investible forest carbon sites to produce a global forest carbon return-on-investment map based on their NPV. We calculated NPV of these returns based on several simplifying assumptions following established values from previous studies [19] . First, we estimated the cost of project establishment at $25 ha −1 . This was based on a wide range of costs that are key to the development of a project, including but not limited to project design, governance and planning, enforcement, zonation, land tenure and acquisition, surveying and research [19] , [36] , [37] . Second, we estimated an annual maintenance cost of $10 ha −1 , which included aspects such as education and communication, monitoring, sustainable livelihoods, marketing, finance and administration [19] , [36] , [37] . Third, we assumed a constant carbon price of $5.8 t −1 CO 2 for the first five years. This price was based on an average price of carbon for avoided deforestation projects recently reported by Forest Trends’ Ecosystem Marketplace [6] (i.e., for the period 2006–2018). After the first five years, we assumed a 5% price appreciation for subsequent years over a project timeframe of 30 years [19] . Based on these criteria, we calculated NPV of annual and accumulated profits over the 30 years, based on a 10% risk-adjusted discount rate. Separately, we repeated the analysis using a range of starting carbon prices, including $1, $5, $10, $15, $25, $50, $100 t −1 CO 2 , based on cost effectiveness thresholds from previous studies [1] . In these analyses, other assumptions remain unchanged, including the project establishment and annual maintenance cost, price appreciation, discount rates and timeframe. Based on these criteria and excluding sites that would be unable to breakeven (i.e., yielding net negative NPVs), we calculated the potential profitable forest areas, as a percentage of the total investible forest areas, associated with these different starting carbon prices. All values of investible carbon and return-on-investment (based on NPV) were summarized to global, regional, and country level estimates (see Table 1 ). For countries that extend beyond tropical latitudes, we only analyze and present data for their tropical extents. These values were rounded to the nearest 1000 values. Uncertainty analyses Stoichiometric factor Previous studies utilized a range of stoichiometric factors, typically ranging between 0.45 and 0.50 [3] , [28] , [29] . We account for this variability by first using a stoichiometric factor of 0.475, which was based on the median value across these reference studies [3] , [28] , [29] . We then repeated the analyses with stoichiometric factors of 0.45 and 0.50 to calculate the respective minimum and maximum values of above and belowground carbon per cell. Root to shoot biomass allometric equations Many site-specific factors can influence the ratio of root to shoot biomass, resulting in variability of the best-fit allometric equations [30] . Here, we account for this variability by utilizing the two allometric equations that best matches global data [30] . This produced two sets of spatially explicit estimates of belowground biomass, from which we calculated the average, minimum and maximum values per cell. Aboveground biomass We incorporated uncertainties, reported at standard deviations, which were inherent to the aboveground biomass dataset [12] . Leakage effects We considered three scenarios of leakage, where the protection of an area of forest results in deforestation beyond its borders to the amounts of 10%, 20%, and 30% of the areas’ carbon volume. This reduces the total investible carbon within each cell, thereby causing a decrease in return-on-investment and the climate mitigation potential within profitable areas to 81.9 ± 51.1, 64.6 ± 40.4 and 48.3 ± 30.3%, or 909.1 ± 567.4, 716.7 ± 448.4, 535.8 ± 336.3 MtCO 2 yr −1 , respectively (Table S1 ). Establishment and maintenance costs We also considered two scenarios of establishment and maintenance cost, where the overall direct cost of protecting areas from deforestation increases by 50% and 100%. We find that this reduces the climate mitigation potential in profitable areas to 80.4 ± 50.4 and 65.7 ± 41.6% or 892.1 ± 559.2 and 728.8 ± 462.2 MtCO 2 yr −1 respectively (Table S1 ). Opportunity costs We also considered the potential for alternative land-use such as agriculture or timber extraction to outcompete the value of protecting forests through carbon financing means. Utilizing agricultural rents (based on 18 crops) and timber value as a proxy for opportunity cost [38] , we excluded areas where opportunity cost exceeds projected net present values. This results in a large decrease in overall climate mitigation potential, almost comparable to the 30% leakage scenario, to 52.3 ± 33.2% or 580.6 ± 368.6 MtCO 2 yr −1 within remaining areas. All analyses were performed in R version 3.6.0 [39] , utilizing the package “raster” for processing and calculations of raster layers [40] . Map visualizations were formed in QGIS [41] . Reporting summary Further information on research design is available in the Nature Research Reporting Summary linked to this article.